Developmentally based scaling of leaf venation architecture explains global ecological patterns Leaf size and venation show remarkable diversity across dicotyledons, and are key determinants of plant adaptation in ecosystems past and present. Here we present global scaling relationships of venation traits with leaf size. Across a new database for 485 globally distributed species, larger leaves had major veins of larger diameter, but lower length per leaf area, whereas minor vein traits were independent of leaf size. These scaling relationships allow estimation of intact leaf size from fragments, to improve hindcasting of past climate and biodiversity from fossil remains. The vein scaling relationships can be explained by a uniquely synthetic model for leaf anatomy and development derived from published data for numerous species. Vein scaling relationships can explain the global biogeographical trend for smaller leaves in drier areas, the greater construction cost of larger leaves and the ability of angiosperms to develop larger and more densely vascularised lamina to outcompete earlier-evolved plant lineages. The angiosperm leaf venation is a developmental marvel, including up to 2 m of length per square centimetre of the leaf, arranged in a regular network. Leaf veins provide mechanical support to display the leaf towards light, and contain the xylem that transports nutrients and water for photosynthesis and transpiration, and the phloem that transports photosynthate and signal molecules from the mesophyll to the rest of the plant [1] . Across species, leaf venation shows enormous structural diversity, the more remarkable because of its shared development and functions. The functional consequences of leaf venation have attracted increasing interest in a widening range of fields, because vein traits, including vein diameters and densities (=length per leaf area), as well as leaf size are key determinants of plant performance and indeed of shifts in the lineages that dominated the world vegetation through deep time [1] , [2] , [3] , [4] , [5] , [6] , [7] , [8] , [9] . Underlying their vascular diversity, angiosperm leaves share a common structural framework and developmental algorithm. Dicotyledonous plants generally possess a reticulate hierarchy based on vein diameter and branching, which evolved early in angiosperms and confers a high transport capacity relative to construction cost [2] , [6] , [9] , [10] , [11] . Typically, the 'major veins' include one or more first order (1°) veins running from the petiole towards the leaf apex, with second order (2°) veins branching off at intervals, and the third order (3°) veins and up to five additional orders of smaller 'minor veins' forming a reticulate mesh between the 1° and 2° veins. General scaling relationships for vascular architecture with leaf size would have far-reaching implications for biogeography, evolution and global ecology. However, despite the strong potential importance of such trends, there have not been any previous conclusive tests for the scaling of vein traits with leaf size across species. Data from three previous studies with ten or fewer species showed a negative scaling of major vein density with leaf size, and minor vein density was independent of leaf size [8] , [12] , [13] . A further study using automated analyses of low-resolution images reported vein density to be independent of leaf size across 339 species [14] ; however, that study measured only a fraction of the vein system and did not distinguish among vein orders [14] and thus, did not allow a conclusive test of general scaling of vein traits. In this study, we made new, high-resolution measurements of vein systems and compiled additional data from the previous literature to create a unique database. We tested developmentally based predictions for the scaling of 10 directly measured key traits and 13 derived key traits (23 traits total), testing each trend for up to 485 globally distributed species, representing 227 genera in 78 families, varying 2,700-fold in leaf area. To our knowledge, this is the most diverse species data set compiled for leaf venation traits. In compiling the database, we included as many families and genera as possible towards maximising species diversity, aiming to determine trends robust across species with leaves that vary widely not only in size, but also in shape and also in texture, in internal and surface anatomy, in rates of photosynthesis and respiration, and in shade and drought tolerance [4] , [15] , [16] . Additionally, we determined whether vein scaling could allow a new method for estimation of intact leaf size from small leaf fragments, which would be valuable given that fossil deposits are rich in fragments, and leaf size can be used as a palaeo-proxy for rainfall and of potential ecosystem biodiversity [7] , [17] , [18] . Finally, we determined the degree that the global scaling of leaf venation with size could be explained on the basis of detailed understanding of leaf anatomy and development during leaf formation and expansion. Global scaling of vascular architecture with leaf size We found strong, global scaling of vascular architecture with leaf size ( Fig. 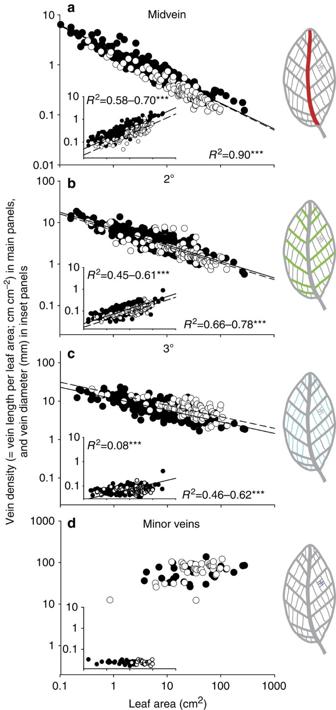Figure 1: Global scaling of leaf venation with leaf size. The scaling of vein density (=vein length/leaf area; main panels) and of vein central diameter (inset panels) for (a) 1°, (b) 2°-, (c) 3°-order veins and (d) minor veins, across a global data set of 485 species of dicotyledons, representing 227 genera from 78 families. Each symbol represents a different species with pinnate venation (that is, with a single 1° vein; filled symbols, solid line) or palmate venation (that is, multiple 1° veins; open symbols, dashed line). Lines were fitted for log (vein density or diameter)=a+blog (leaf area). The scaling of vein traits with leaf area becomes shallower from 1° to 2° to 3° veins, and minor vein diameter and density are independent of leaf size, as predicted from the developmental model. Significance of fitted lines: ***P<0.001. 1 ; Table 1 ). These trends were robust across the full range of leaf sizes (leaf area ranging from <1 to 280 cm 2 ; Supplementary Table S1 , Supplementary Data 1 ), though our sampling included more small leaves than large leaves, reflecting the greater commonness of smaller leaf sizes globally [7] . Indeed, the trends were so strong that subsampling of species showed the same relationships, that is, within the given genera and families (Methods). Overall, the major veins showed strong positive scaling in vein diameters and negative scaling in vein density with leaf size, with the magnitude of scaling slopes (that is, b in trait= a ×leaf area b ) declining from 1° to 2° to 3° veins, and the minor veins showed no significant scaling of vein densities or diameters with leaf size. Thus, the midvein diameter increased close to geometrically with leaf size ( b =0.45; 95% confidence interval (CI) 0.43, 0.48), the 2° vein diameter less than geometrically ( b =0.37; 95% CI 0.34, 0.39) and the 3° diameter only weakly (only for pinnately veined species; b =0.22; 95% CI 0.20, 0.25). The 1° and 2° vein densities declined close to geometrically ( b =−0.40 to −0.53; 95% CI −0.38, −0.57) and the 3° vein density declined conservatively with leaf size ( b =−0.30; 95% CI −0.28, −0.32). By contrast, the diameters and density of minor veins were independent of leaf size as was the total vein density, because minor veins typically accounted for the bulk of total vein length (on average 84%; Supplementary Table S1 ). The trends in vein diameters and densities drove additional scaling of the vein cross-sectional area and projected area, and of the vein volume ( Table 1 ). Notably, the total vein volume per leaf area, which would contribute to leaf construction cost [19] , [20] , increased with leaf size less than geometrically. These scaling relationships for vein diameters and densities were strong, despite the wide species variation in cell and leaf structure, physiology and ecology. Figure 1: Global scaling of leaf venation with leaf size. The scaling of vein density (=vein length/leaf area; main panels) and of vein central diameter (inset panels) for ( a ) 1°, ( b ) 2°-, ( c ) 3°-order veins and ( d ) minor veins, across a global data set of 485 species of dicotyledons, representing 227 genera from 78 families. Each symbol represents a different species with pinnate venation (that is, with a single 1° vein; filled symbols, solid line) or palmate venation (that is, multiple 1° veins; open symbols, dashed line). Lines were fitted for log (vein density or diameter)= a + b log (leaf area). The scaling of vein traits with leaf area becomes shallower from 1° to 2° to 3° veins, and minor vein diameter and density are independent of leaf size, as predicted from the developmental model. Significance of fitted lines: *** P <0.001. Full size image Table 1 Parameters for the scaling of vein traits with leaf size. Full size table Estimating intact leaf size from venation in leaf fragments A second major finding of our study was a unique application of these vein-scaling relationships for accurately predicting leaf size from small leaf subsamples ( Fig. 2 ). Leaf size was correlated with the 2° vein density measured in rectangles sampled midway between midvein and margin, centrally in the top, middle and bottom third of the leaf, or centrally in the leaf alongside the midvein ( r =−0.83 to −0.86). These relationships follow from the negative scaling of whole-leaf 2° vein density with leaf size ( Fig. 1b ), because the 2° vein density measured on subsamples was strongly correlated with that determined from the whole leaf (log-transformed data; r= 0.82–0.87; P <0.001). This relationship would allow estimation of the intact leaf size from fossil fragments. An equation was determined for estimating the leaf size from subsampled regions of central leaf lamina, based on the 2° vein density ( Fig. 2 ): log (leaf area)=1.96–2.04×log (subsample 2° vein density) ( R 2 =0.80; P <0.001). For estimation based on a subsampled region of lamina adjacent to the midvein, which would enable the 2° veins to be decisively located (that is, from fragments including the midvein), log (leaf area)=1.62–1.82×log (subsample 2° vein density) ( R 2 =0.74; P <0.001). These trends enable the estimation of intact leaf size from fossil fragments to improve resolution of leaf size, and potential palaeo-estimation of rainfall and of potential ecosystem biodiversity [7] , [17] , [18] . 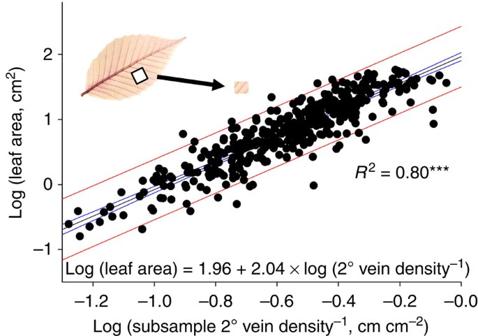Figure 2: Estimating intact leaf size from venation in leaf fragments. Leaf size predicted from the density of 2° veins (=vein length per leaf area) in subsampled leaf regions across a global leaf data set of 386 dicotyledonous species. The subsampled regions contained at least two 2° veins and had mean size ± s.e. of 0.27 cm2± 0.0015. This relationship can allow the determination of leaf size from fragments. The 95% confidence intervals are in blue and 95% prediction intervals in red58, equivalent to,, andfor estimates based on 5, 10 and 20 leaf fragments. Figure 2: Estimating intact leaf size from venation in leaf fragments. Leaf size predicted from the density of 2° veins (=vein length per leaf area) in subsampled leaf regions across a global leaf data set of 386 dicotyledonous species. The subsampled regions contained at least two 2° veins and had mean size ± s.e. of 0.27 cm 2 ± 0.0015. This relationship can allow the determination of leaf size from fragments. The 95% confidence intervals are in blue and 95% prediction intervals in red [58] , equivalent to , , and for estimates based on 5, 10 and 20 leaf fragments. Full size image Synthetic model for developmentally based leaf vein scaling A third major finding of our study is the explanation of these scaling relationships from a global developmental algorithm. We developed a new synthetic model for the development of vein hierarchy from apical, marginal and plate meristems, based on previously published information for vein development in model species Arabidopsis [21] , [22] , [23] , [24] , [25] , [26] , [27] , [28] ( Fig. 3 ), which we further confirmed for 27 other dicotyledon species of a wide range of leaf form on the basis of 25 earlier studies ( Supplementary Table S2 ). This developmental algorithm leads automatically to the global scaling trends in Figs 1 and 2 , and Table 1 . In early leaf development, the primordium, formed by apical and marginal meristems, undergoes a 'slow' limited expansion phase, principally because of cell proliferation, and a 'rapid' dramatic expansion phase, mainly because of cell expansion, though cell divisions continue ( Fig. 3a ). The vein orders form in overlapping sequence, beginning with vascular identity gene expression and signal transduction in ground meristem, followed by the differentiation of procambium and finally vein maturation ( Fig. 3b ). The 1° and 2° veins are formed during the slow phase, the 3° veins next, and the minor veins principally during the rapid phase. The initiation of procambial strands for each vein order is limited by the need to maintain a critical cell number or distance between new strands and the duration that the ground meristem can perceive vascular-forming signals. While procambial strands differentiate into vascular tissue and vascular tissues mature, these nascent veins can extend during ongoing leaf expansion. Thus, the vein densities of each order peak as procambium forms and then decline as leaf expansion pushes veins apart, but the minor vein density stabilises as their initiation is maintained during leaf expansion ( Fig. 3c ). Finally, the 1° and 2° veins have prolonged diameter growth, whereas 3° veins and minor veins rapidly attain maximum diameter ( Fig. 3d ). 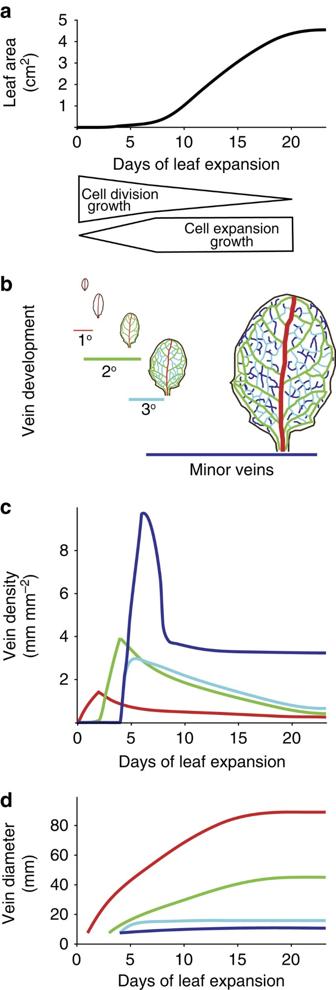Figure 3: Synthetic model for leaf expansion and vein development. This model was developed from data forArabidopsisleaves21,22,23,24,25,26,27,28and 27 other dicotyledonous species. (a) The primordium, formed by apical and marginal meristems, undergoes a 'slow' limited expansion phase, principally because of cell proliferation, and a 'rapid' dramatic expansion phase, mainly because of cell expansion, though cell divisions continue. (b) Vein orders form in overlapping sequence, beginning with vascular identity gene expression and signal transduction in ground meristem, followed by the differentiation of procambium, and finally vein maturation. The 1° and 2° veins are formed during the slow phase, the 3° veins next, and the minor veins principally during the rapid phase. The procambial strands initiated for each vein order are limited by the need to maintain a critical cell number or distance between new strands and the duration that the ground meristem can perceive vascular-forming signals. (c) Vein densities of each order peak as procambium forms, then decline as leaf expansion pushes veins apart, but the minor vein density stabilises as vein initiation is maintained during leaf expansion. (d) The 1° and 2° veins have prolonged diameter growth, whereas 3° veins and minor veins rapidly attain maximum diameter. Although a few additional 2° veins form later in development, this affects only a minority of the mature vein system. Figure 3: Synthetic model for leaf expansion and vein development. This model was developed from data for Arabidopsis leaves [21] , [22] , [23] , [24] , [25] , [26] , [27] , [28] and 27 other dicotyledonous species. ( a ) The primordium, formed by apical and marginal meristems, undergoes a 'slow' limited expansion phase, principally because of cell proliferation, and a 'rapid' dramatic expansion phase, mainly because of cell expansion, though cell divisions continue. ( b ) Vein orders form in overlapping sequence, beginning with vascular identity gene expression and signal transduction in ground meristem, followed by the differentiation of procambium, and finally vein maturation. The 1° and 2° veins are formed during the slow phase, the 3° veins next, and the minor veins principally during the rapid phase. The procambial strands initiated for each vein order are limited by the need to maintain a critical cell number or distance between new strands and the duration that the ground meristem can perceive vascular-forming signals. ( c ) Vein densities of each order peak as procambium forms, then decline as leaf expansion pushes veins apart, but the minor vein density stabilises as vein initiation is maintained during leaf expansion. ( d ) The 1° and 2° veins have prolonged diameter growth, whereas 3° veins and minor veins rapidly attain maximum diameter. Although a few additional 2° veins form later in development, this affects only a minority of the mature vein system. Full size image Given this developmental algorithm is general, vein diameters and densities should show specific power-law scaling with leaf size across species ( Supplementary Table S3 ). The 1° vein diameter would increase close to geometrically with increasing leaf size as thickening growth can continue during most of the leaf expansion, whereas 2° and 3° vein diameters would increase conservatively with leaf size, and minor vein diameters would be independent of leaf size. The densities (length/leaf area) of the major veins should show declines in larger leaves. The 1° and 2° vein densities would decline geometrically with increasing leaf size, given they are formed in limited quantities during the slow expansion phase and are then pushed apart during subsequent rapid expansion. We note that despite even moderate changes in cell size or cell number between initiating procambial strands within or across species, the negative scaling of 1° and 2° vein densities with final leaf size would still approach geometric. For example, even if the cell number between the procambial strands were to double or triple (that is, the distance between initiating procambial strands were to double or triple), because the expansion of the leaf is many 1,000-fold, the final 1° and 2° vein densities would still decline close to geometrically. The 3° vein density should decline more weakly, given these veins are formed later, and thus pushed apart less in the ongoing leaf expansion. Notably, these trends for the decline of major vein densities with leaf size could be modified by increasing or decreasing the initiation of veins, or their relative trajectories, or changing the shape of the leaf with size ( Fig. 4 ). However, changes in vein initiation would likely have only slight effects on the global scaling of major veins with leaf size, because such initiation is limited by space and time in the slow phase of leaf expansion, and these veins are subsequently pushed apart. Further, additional major veins can also be formed by modification of the smaller veins later in leaf development, but this affects only a minority of the mature vein system [22] . 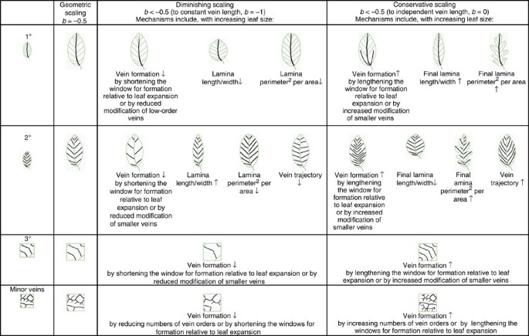Figure 4: The geometric scaling of vein density with leaf size expected because of leaf expansion and mechanisms for its modification. The first column shows vein orders, and the three columns to the right show scenarios for the scaling of their vein density (=vein length/leaf area) with leaf size. According to the baseline expectation of geometric similarity, in which traits scale with size based on their dimensionality as a length, area or volume (for example, vein length scales with leaf area0.5, and thus vein density with leaf area−0.5), veins are spaced out proportionately with increasing leaf size, given no change in the numbers of veins initiated, in their relative trajectories, or in the shape of the leaf. If vein density declines more than under geometric scaling, this is indicated as 'diminishing scaling' andb<−0.5; with an extreme scenario being independent vein length across a gradient of leaf sizes, withb=−1. Diminishing scaling would occur if larger leaves have fewer veins initiated, or if larger leaves shift in shape (for example, in length/width ratio, or edge complexity, that is, perimeter2per area), or if vein trajectory changes, either because of changes in procambium development, or later changes in the relative expansion of lamina in different areas of the leaf. If the vein density decreases less than expected under geometric scaling, this is indicated as 'conservative scaling' andb>−0.5; with an extreme scenario being independent vein density, in whichb=0. This pattern could arise in the opposite set of conditions as for diminishing scaling. Figure 4: The geometric scaling of vein density with leaf size expected because of leaf expansion and mechanisms for its modification. The first column shows vein orders, and the three columns to the right show scenarios for the scaling of their vein density (=vein length/leaf area) with leaf size. According to the baseline expectation of geometric similarity, in which traits scale with size based on their dimensionality as a length, area or volume (for example, vein length scales with leaf area 0.5 , and thus vein density with leaf area −0.5 ), veins are spaced out proportionately with increasing leaf size, given no change in the numbers of veins initiated, in their relative trajectories, or in the shape of the leaf. If vein density declines more than under geometric scaling, this is indicated as 'diminishing scaling' and b <−0.5; with an extreme scenario being independent vein length across a gradient of leaf sizes, with b =−1. Diminishing scaling would occur if larger leaves have fewer veins initiated, or if larger leaves shift in shape (for example, in length/width ratio, or edge complexity, that is, perimeter 2 per area), or if vein trajectory changes, either because of changes in procambium development, or later changes in the relative expansion of lamina in different areas of the leaf. If the vein density decreases less than expected under geometric scaling, this is indicated as 'conservative scaling' and b >−0.5; with an extreme scenario being independent vein density, in which b =0. This pattern could arise in the opposite set of conditions as for diminishing scaling. Full size image In contrast with the major venation, by the developmental model, the minor vein density is expected to be independent of leaf size across leaves globally. This is enabled by the ongoing formation of minor vein orders during the extended rapid phase of leaf expansion ( Fig. 3c ). Notably, unlike in Arabidopsis ( Fig. 3 ), in many species, substantial leaf expansion continues after all the vein procambium is formed, and minor vein density declines as leaves continue to expand [29] , [30] . However, even among such species, this effect does not drive a general negative scaling of the minor vein density with increasing final leaf size, because the developmental model allows changes in timing or extent of the minor vein initiation relative to leaf expansion throughout the rapid phase of leaf expansion, or increases in the number of minor vein orders ( Fig. 4 ). Thus, it would be possible to achieve higher final minor vein density in a smaller leaf by limiting leaf expansion after all veins are formed; or higher final minor vein density without change in leaf size by compensating with increasing expansion before the final vein order is formed; or higher final minor vein density with a larger leaf, with still greater expansion before the final vein order is formed; or a larger leaf without change in minor vein density by increasing expansion only before the final vein order is formed, thus initiating veins in the same proportion to leaf area as in the small leaf. All of these scenarios can occur, for example, for the sun relative to shade leaves of given species, and across populations or across closely related species adapted across habitats [4] , [12] , [30] , [31] , [32] , [33] , [34] , [35] , [36] , [37] . Notably, leaf expansion relative to vein formation can be influenced by modulating cell proliferation, which especially affects expansion before the final vein order is formed, and final cell size, which mainly affects expansion after all veins are formed [38] , [39] . Changes in vein density independently of leaf size can also be evolved by maintaining the same leaf expansion, but increasing or reducing the number of vein orders [30] . In sum, unlike the major veins, which are formed in the early slow expansion phase, the minor veins, being formed throughout the rapid expansion phase, can in principle develop to a wide range of final vein densities in the mature leaf, independently of the final leaf size. Empirical support for developmentally based leaf vein scaling The developmentally based expectations for the scaling of venation architecture ( Supplementary Table S3 ) were consistent with the global trends for all 23 traits tested ( Fig. 1 and Table 1 ). The developmental algorithm would result in the greater vein diameter of 1° and 2° veins in larger leaves and lower vein densities for all orders of major veins in larger leaves ( Fig. 5 ). The quantitative expectations derived from the developmental algorithm were constrained power-law exponents (for example, '±20%') rather than specific exponents, reflecting the reality of the developmental mechanism and structural variation. Notably, the global scaling trends of major vein densities were robust to shifts in other traits with leaf size, that is, weak increases in 1° and 2° vein numbers and widening of leaf shape in larger leaves ( Supplementary Table S4 ). 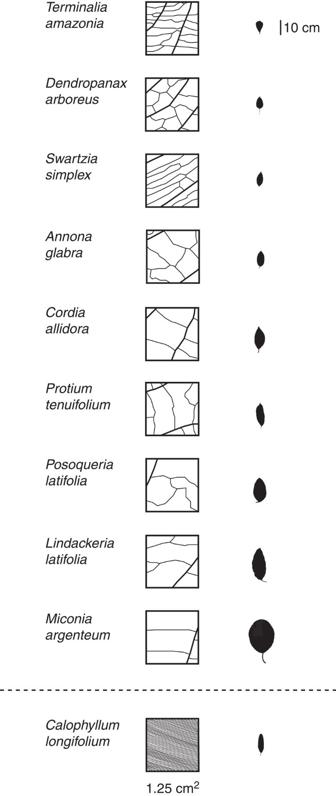Figure 5: General decline of major vein density with increasing leaf size. The trend observed across species for the Panamanian rainforest trees. The micrograph drawings are traces of regions of the lamina with 2° and 3° veins, matched with leaf silhouettes for given species, all to the same scale, thus showing the greater spacing between major veins in larger leaves. Minor veins (not shown) do not show correlation of spacing or scaling with leaf size across species. TheCalophyllum longifoliumleaf has exceptional venation, with parallel 2° veins branching from the midvein and transverse 3° veins. This rare exception shows that the general venation-scaling pattern, so typical across species, can be broken, given very strongly different venation development. ForCalophyllum, the 2° veins development shows similarity to that of minor veins in typical dicotyledonous leaves (seeSupplementary Table S2). Figure 5: General decline of major vein density with increasing leaf size. The trend observed across species for the Panamanian rainforest trees. The micrograph drawings are traces of regions of the lamina with 2° and 3° veins, matched with leaf silhouettes for given species, all to the same scale, thus showing the greater spacing between major veins in larger leaves. Minor veins (not shown) do not show correlation of spacing or scaling with leaf size across species. The Calophyllum longifolium leaf has exceptional venation, with parallel 2° veins branching from the midvein and transverse 3° veins. This rare exception shows that the general venation-scaling pattern, so typical across species, can be broken, given very strongly different venation development. For Calophyllum , the 2° veins development shows similarity to that of minor veins in typical dicotyledonous leaves (see Supplementary Table S2 ). Full size image A rare exception to the global scaling trends was found in the case of Calophyllum longifolium ( Fig. 5 ), which had exceptional venation, with parallel 2° veins branching from the midvein and transverse 3° veins. For Calophyllum , the development of 2° veins shows similarity to that of minor veins in typical dicotyledonous leaves ( Supplementary Table S2 ). This rare exception shows that the venation-scaling patterns that are so general across dicotyledons can be broken, given very strongly different venation development. The matching of global trends with developmental basis provides powerful new explanation for the trends of vascular architecture with leaf size across species. We present key discoveries in leaf structure and function. The most important finding was the extremely strong, global scaling of leaf venation architecture with leaf size. These relationships provide new fundamental understanding of leaves with potential global scale impacts on leaf ecology, plant carbon economy and drought tolerance, and the history of vegetation worldwide through deep time. We described not only new venation architecture scaling trends, but also a powerful new application for estimating intact leaf sizes from leaf fossil fragments, which would improve estimation of climates in the deep past from the fossil floras, and a developmental mechanism that explains these relationships. The generality across species of the developmental programme presented, synthesised from previous work, is striking, and is consistent with genetic obstacles to evolution of vein traits and redundant developmental pathways [23] , [40] . Indeed, auxin signalling and gene expression patterns during vein development are conserved in different species [41] , [42] . Our confirmation of the major steps in leaf and vein development across species compiled in Supplementary Table S2 indicates that the developmental mechanisms and growth dynamics previously established for Arabidopsis are general across a wide range of dicotyledons, as had been implicitly assumed in the studies of this model species. Further, the contrasting scaling of the major and minor vein systems shown here is consistent with deep disjuncts in numerous other features of major and minor veins across angiosperms, including their procambial anatomy and development, genetic programmes, xylem and phloem function, and plasticity and evolution across environments ( Supplementary Table S5 ). Although the global trends could be explained quantitatively on a developmental basis according to the synthetic model presented, we note that these trends would be reinforced by additional functional selection, that is, by adaptation in structure and physiology to the environment. For example, when a larger leaf is selected for a given ecological advantage, this would reinforce the global scaling trends, because that leaf would have a lower major vein automatically, according to the developmental mechanism. Additionally, this larger leaf would require a larger midrib for biomechanical and hydraulic support, and that would arise from the linked development of midrib diameter and leaf size. Further, selection for higher or lower minor vein density, independently of the final leaf size, would reinforce the overall global independence of the minor vein density from the leaf size. Indeed, the minor vein density is a key determinant of leaf hydraulic capacity and photosynthetic rates, and there would be strong benefit in an ability to vary across a wide range of environments, independently of leaf size [3] , [4] , [6] , [43] . The scaling relationships and their developmental basis have unique and key implications for biogeography, physiological adaptation, palaeobiology and vein network theory. The general linkage of major vein density with leaf size provides a mechanism to explain perhaps the most famous of global plant biogeographical trends, the predomination of small leaves in drier and more exposed habitats [7] , [44] . Indeed, the variation in leaf size across environments varying in moisture has appeared in the literature going back to Theophrastus, von Humboldt and Raunkiaer [45] . Classically, this trend has been attributed to an indirect advantage of small leaves in reducing overheating, given thinner boundary layers and more rapid convective cooling [45] , [46] . However, the scaling of major vein density provides a direct, hydraulically based mechanism. Modelling and experiments showed that such higher major vein density in smaller leaves in principle provides redundant 'superhighways' for water transport that contribute to drought tolerance by routing water around blockages caused by drought-induced xylem embolism, and additionally protect the hydraulic system from vein damage [8] , [13] . Another implication of the global scaling is that larger leaves, with greater major vein diameters and greater vein volume per area, intrinsically have larger vascular costs. Notably, the total vein volume per leaf area increases less than geometrically with leaf size, leading to a lower increase than would be obtained from a non-hierarchical system with uniform scaling behaviour. Nonetheless, the increase of vein volume per area would contribute importantly in the general decline of photosynthetic leaf area per investment of carbon in larger leaves [19] , [20] . However, despite their greater drought sensitivity and greater carbon cost per photosynthetic surface, large simple leaves are known to be highly competitive in resource-rich environments [5] , [9] , [44] . The developmental algorithm and scaling relationships we have shown makes this possible for dicotyledons, providing a strong ecological advantage. Dicotyledons can produce large leaves with both large major veins for mechanical support and high vein densities that enable transpirational cooling and high photosynthetic rates [1] , [47] , [48] , [49] . Large simple leaves with high vein density are an angiosperm innovation, because the ongoing production of minor veins in expanding leaves depends on the plate meristem that is typically found only in angiosperms [18] . With few exceptions, in earlier-derived plant lineages, such as ferns and gymnosperms, even small leaves (or leaflets or pinna) cannot achieve high vein densities, lacking the capacity to form small-diameter minor veins, [18] and greater leaf expansion would push earlier-formed veins yet further apart. Thus, large pinnae in those species would inevitably have low vein densities, and not only lack high gas exchange rates, but would be potentially inviable in high irradiance environments, without the water transport capacity to cool the leaves. Notably, the dicotyledon developmental programme allows for not only large, competitive leaves, but a dramatic range of leaf sizes with a wide spectrum of total vein densities and photosynthetic rates [16] . For example, a large leaf may be selected for a plant of a moist area, for effective light capture and photosynthesis relative to biomass allocation [44] , and a small leaf may be selected in drought-tolerant species [8] ; both may have high minor vein densities, enabling high photosynthetic rates when water is available. The potential of angiosperms to vary strongly in vein density enables dominance in a far greater range of habitats than other plant lineages [3] , [6] , [48] , especially as leaf size can adapt independently to optimise other ecological benefits against costs [6] , [7] , [44] . Our findings extend the empirical basis and theory of vein network scaling by providing high-resolution data, novel global trends and explicit integration of the development and function of the vein-order hierarchy. A recent study used low-resolution automated measurements of leaf images and measured vein segments without considering the vein-order hierarchy, and found no vein trait to scale with leaf size for 339 species [14] . Notably, the independence of total vein density from leaf size in that study was not a property of the venation, but reflected the low-measurement resolution having been uniformly applied across all leaf sizes ( Fig. 6 ). That study also presented exponential and power-law frequency distributions of vein segment lengths and diameters within given leaves, but a previous, higher resolution study demonstrated a unimodal skewed distribution for vein segment diameters [50] . Notably, the theoretical interpretation of vein scaling is greatly improved by explicit consideration of the vein-order hierarchy and the details of its development. Price et al . [14] proposed that vein scaling arises because 'growing veins stop and/or branch at random with a constant probability per unit length', but the patterns in fact emerge from a developmental algorithm with highly regulated sequence and directionality ( Fig. 3 ) [24] , [25] , [42] . Price et al . [14] proposed that 'the constraints of mass flow require vein radii to connect hierarchically in a way that is scale-free (fractal-like)', but individual vein segments are not necessarily connected hierarchically, that is, from large to small; rather, segments of all diameters are interconnected in the reticulate network. Instead the hierarchical organisation is at the level of vein orders, and this hierarchy has indeed been found to reduce construction cost relative to flow capacity [6] . Finally, Price et al . [14] proposed that vein density should be independent from leaf size, because a constrained distance between the minor veins and thus a high vein density is needed for water and sugar transport. This idea comes from physiological studies that showed such an importance of high vein density but also adaptive variation across species [4] , [43] , [51] , [52] , [53] . Indeed, we found here a considerably higher and more variable range of values for total vein density ( Fig. 6 ). However, this importance of vein density alone is not sufficient to explain the independence of total vein density from leaf size. The developmental algorithm provides a basis for that pattern, as it enables independent evolutionary optimisation of total vein density and leaf size along separate ecological axes. 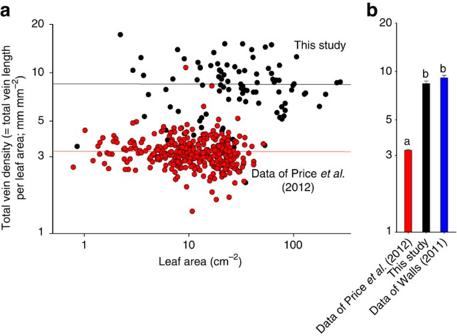Figure 6: Independence of total vein density from leaf size and the importance of high-resolution measurement of the leaf venation architecture. (a) Independence of total vein density (=vein length per leaf area) from leaf size across the global database for dicotyledonous species in this study (black points) and in a previous study by Priceet al.14that used automated measurements on low-resolution images of cleared leaves (red points). Values for vein density are higher on average and show greater variation among species when determined using high resolution (note log scale). (b) Mean±s.e. for total vein density from this study (black bar) with that of Priceet al. (red bar) and that of Walls49for 111 diverse dicotyledonous species (blue bar), which focused only on vein density and not on leaf size. The mean value of Priceet al. was three-fold lower than those for this study and Walls (P<0.001), and the s.d. of the data of Priceet al. was three-fold lower than those of this study and Walls (0.78 relative to 3.06 and 3.26, respectively;P<0.001;F-ratio test). Our data were not significantly different from those of Walls (as indicated by the same lowercase letters), but the low values for vein density of Priceet al. suggest that the pattern shown arose from the independence of their low measurement resolution from leaf size. Figure 6: Independence of total vein density from leaf size and the importance of high-resolution measurement of the leaf venation architecture. ( a ) Independence of total vein density (=vein length per leaf area) from leaf size across the global database for dicotyledonous species in this study (black points) and in a previous study by Price et al . [14] that used automated measurements on low-resolution images of cleared leaves (red points). Values for vein density are higher on average and show greater variation among species when determined using high resolution (note log scale). ( b ) Mean±s.e. for total vein density from this study (black bar) with that of Price et al . (red bar) and that of Walls [49] for 111 diverse dicotyledonous species (blue bar), which focused only on vein density and not on leaf size. The mean value of Price et al . was three-fold lower than those for this study and Walls ( P <0.001), and the s.d. of the data of Price et al . was three-fold lower than those of this study and Walls (0.78 relative to 3.06 and 3.26, respectively; P <0.001; F -ratio test). Our data were not significantly different from those of Walls (as indicated by the same lowercase letters), but the low values for vein density of Price et al . suggest that the pattern shown arose from the independence of their low measurement resolution from leaf size. Full size image In conclusion, the vein scaling relationships increase the core understanding of the structure and function of leaves that has global implications for leaf distribution, plant drought tolerance, carbon economy and the history of vegetation worldwide through deep time. We also introduced a powerful new application for estimating intact leaf sizes from leaf fossil fragments, which would improve estimation of climates in the deep past from fossil floras. Our three major findings (novel global trends, novel application to predicting leaf size from tiny fragments and explanation of trends by a general developmental mechanism) represent distinctive and major advances over earlier work. Leaf anatomy and developmental algorithms have substantial impacts on global biogeography and deep time evolution. Once discerned, the simplicity of these linkages highlights the fascinating beauty and far-reaching impacts of the development of leaf venation, and can serve to initiate researchers in a wide range of fields as well as laypeople into the importance and applications of knowledge of leaf venation architecture. Collecting data and compiling the global database A global data set was compiled for up to 23 vein traits for 485 dicotyledon species, representing 227 genera from 78 families. Virtually all data were based on original measurements of chemically cleared leaves, supplemented with previously published data ( Supplementary Methods and Supplementary Table S6 ). Leaf clearing All leaf clearing used the same protocol as previously published by the authors [4] , [8] , [12] , [54] , [55] . Briefly, leaves were fixed in 70% formalin–acetic acid–alcohol (48% ethanol: 10% formalin: 5% glacial acetic acid: 37% water) and cleared in 2.5–5% sodium hydroxide in water or ethanol followed by sodium hypochlorite bleach, and stained with safranin and fast green. Analyses of images of vein systems All measurements of vein traits (>600 leaves in this study) were made manually from images of chemically cleared leaves. We did not use automated vein measurement software, though a recently published study used such a programme to analyse images for 339 dicotyledon leaves [14] . As recognised by that study's authors, that approach resulted in low-resolution measurements of an unspecified fraction of the vein density: 'Note that our values for network density overlap with, but are generally lower than those reported for leaves imaged under [high] magnification. We suspect that these differences are due to the fact that our images are unmagnified photographs, which may not resolve all of the very smallest veins, yet which include all major veins.' Notably, those unresolved 'very smallest veins', that is, minor veins, make up the bulk of the length of the leaf venation ( Fig. 6 ; Supplementary Table S1 ). Thus, we used manual measurements to ensure accuracy and resolution of all the veins, and further to distinguish the different scaling behaviours of the major veins and minor veins. Species virtually all had three orders of major veins and three or more orders of minor veins. Leaves were assessed as palmately veined if more than one vein branched from the petiole with >75% the diameter of the midvein. The 2° veins were defined as those that branched from the 1° veins, distinct in size and pattern from the 3° veins, which formed the largest-gauge reticulate mesh in the leaf. We note that despite this well-accepted vein classification paradigm [10] , [11] , there is a degree of uncertainty in categorising vein orders in the mature leaf, especially in distinguishing 3° veins from the smaller 2° veins or from larger 4° veins. Vein diameter alone cannot be used to categorise vein orders, as vein diameters vary continuously in the whole leaf [50] , but partitioning veins by including information of branching order is practicable. In the 2° veins, we included the so-called 'minor' 2° veins (that is, 'intersecondary 2° veins'), which are shorter in length and branch between typical 2° veins. Because of its atypical venation ( Fig. 5 ), Calophyllum longifolium was not included in the analyses of 2°, 3° or major veins. For the original data collected for the database, measurements were made for leaf size and shape, and major vein traits on scans or images of whole leaves. Cleared and stained leaves were digitally scanned at 600–1200 dpi (Epson Perfection 3170 or 4490 Photo, Epson America Inc., Long Beach, CA, USA), and analysed with Image J software [56] . Whole, cleared leaf images were measured for leaf area, maximum leaf length: width as an index of shape, numbers of 1° and 2° veins, and diameters and lengths of 1°, 2° and 3° veins. Densities of minor veins were determined from one to two subsampled regions of 1.5–1.9 mm 2 taken centrally on the right-hand side of each leaf, imaged at ×5–40 magnification using light microscopy (Zeiss compound microscope, Zeiss, Germany; with Nikon Coolpix 4500 digital camera, Nikon, Tokyo, Japan; or Leitz DMRB microscope, Leica Microsystems Inc., Bannockburn, IL, USA; with a SPOT Insight 4 Mp Mosaic 14.2 camera and SPOT software v. 4.6, Diagnostic Instruments, Inc., Sterling Heights, MI, USA). Measured vein diameters included the lignin-stained portions (xylem and fibres). The diameters of 1° and central 2° veins were measured halfway along their length, perpendicular to the vein. For the Axelrod data set, the 3° vein diameters were measured from the whole-leaf scans from the centre of four segments centrally in the leaf; for the other data sets, vein diameters were measured in the centre of two or more vein segments for 3° veins and veins of higher orders from the microscope images. Vein lengths were measured for all 1° veins, and for 2° veins on one half of the leaf, and doubled for total 2° vein length. The density of 3° veins was averaged for one to three subsampled regions measured centrally in the top, middle and bottom thirds of the right side of the leaf. Densities of higher-order veins were determined from the microscope images. Total vein density was determined as the sum of 1°, 2°, 3° and minor vein densities. For each vein order, the vein cross-sectional surface area per leaf area was estimated by multiplying the vein density by π×the vein diameter. The vein-projected area per leaf area (that is, the proportion of leaf lamina obstructed by vein) was determined by multiplying the vein diameter by vein density. Vein volume per leaf area was determined by multiplying the vein density by π× the square of half the diameter. Vein surface areas and volumes for major veins were determined by summing for the 1°, 2° and 3° veins. Proportional major vein allocation to given orders was calculated for vein lengths, areas and volume by dividing the value for a vein order by that for the whole major vein system. Overall proportional major and minor vein allocation were determined by dividing by the values for the total vein system. Using the Axelrod data set, we determined the degree that the leaf area could be predicted from 2° vein density measured in small rectangle subsections ( n= 386 species). The rectangles were drawn to include at least two 2° veins. For each leaf, we subsampled four rectangular boxes. The first three boxes were intended to represent typical fragments and were located in the top, middle and bottom thirds of the leaf between the midvein and margin, and ranged from 0.002 to 3 cm 2 , on average 0.3 cm 2 (on average 3% of leaf area). Because our ability to identify 2° veins in subsampled areas might have been unrealistically simple given our ability to see the whole cleared leaf, we additionally considered an approach in which the 2° veins might be more difficult to identify within a fragment. Thus, a fourth rectangle was subsampled, which was alongside the midvein centrally in the leaf and which included at least two 2° veins. Such a practice could be used to estimate the leaf size from those fragments that include the midvein, and for which the branching 2° veins can be identified unquestionably. Determination of scaling relationships Scaling relationships among traits were determined by fitting lines to log-transformed data, thus modelling the relationships of vein traits as power-law functions of leaf area: trait= a ×leaf area b . Power-law scaling was expected given that traits have proportional relative growth rates in development, or proportional relative shifting across species [57] . Geometric scaling predictions were derived [57] by treating each fundamental trait as a length ( L ), area ( A ) or volume ( V ), where A L 2 and V L 3 . Thus, vein diameter is an L A 0.5 ; vein density is an L / A A −0.5 ; vein surface area per leaf area is an A / A A 0 , and vein volume per leaf area is a V / A A 0.5 . For an analysis robust to outliers, for all relationships, the non-parametric Spearman's correlation coefficient ( r s ) was tested first [58] , and if not significant at P =0.05, then no relationship was concluded. If r s was significant, we followed a previous study [14] in using standard major axes or ordinary linear regression for fitting lines, depending on the calculation of the given trait and thus, its relative level of measurement error (using SMATR [59] ), and tested the relationship of each area-normalised trait with leaf area for spurious correlation (see Supplementary Methods ). In determining trends across species, we focused on historical scaling analyses rather than phylogenetically controlled comparisons, consistent with our aim to determine general scaling arising from a shared developmental constraint. Notably, genus-by-genus analyses produced comparable patterns, as did phylogenetically controlled tests within lineages for Acer , Plantago and Viola for which highly resolved phylogenetic trees were available (unpublished data) [12] . However, we note that the scaling trends within given lineages may depart from the global across-species trends shown here, especially in lineages adapted across environments. For example, frequently, species within a genus adapted to drier or more exposed conditions will have smaller leaves with higher minor vein densities, resulting in a slight negative scaling of minor vein density with leaf size. Such scaling differs from the more general baseline developmental model and scaling relationships shown here. Thus, even though the negative correlation of minor leaf venation with leaf size in such lineages emerges from a coordinated developmental process, it is not intrinsically necessary, but apparently aries because of the two traits being coselected during adaptation for a given environment, a type of 'concerted convergence' of traits that could otherwise be unlinked [60] . Vein development and its plasticity and adaptation across environments are further discussed in Supplementary Table S5 . How to cite this article: Sack, L. et al . Developmentally based scaling of leaf venation architecture explains global ecological patterns. Nat. Commun. 3:837 doi: 10.1038/ncomms1835 (2012).